TRIP13 promotes error-prone nonhomologous end joining and induces chemoresistance in head and neck cancer Squamous cell carcinoma of the head and neck (SCCHN) is a common, aggressive, treatment-resistant cancer with a high recurrence rate and mortality, but the mechanism of treatment resistance remains unclear. Here we describe a mechanism where the AAA-ATPase TRIP13 promotes treatment resistance. Overexpression of TRIP13 in non-malignant cells results in malignant transformation. High expression of TRIP13 in SCCHN leads to aggressive, treatment-resistant tumors and enhanced repair of DNA damage. Using mass spectrometry, we identify DNA-PKcs complex proteins that mediate nonhomologous end joining (NHEJ), as TRIP13-binding partners. Using repair-deficient reporter systems, we show that TRIP13 promotes NHEJ, even when homologous recombination is intact. Importantly, overexpression of TRIP13 sensitizes SCCHN to an inhibitor of DNA-PKcs. Thus, this study defines a new mechanism of treatment resistance in SCCHN and underscores the importance of targeting NHEJ to overcome treatment failure in SCCHN and potentially in other cancers that overexpress TRIP13. Squamous cell carcinoma is a common cancer occurring in the head and neck, skin, oesophagus, lung and cervix. Squamous cell carcinoma of the head and neck (SCCHN) is the sixth most common cancer globally [1] . Half of the 600,000 patients diagnosed annually will die in 5 years [1] , [2] . The morbidity is worse than breast cancer or melanoma [2] because of late diagnosis and tumor relapse. Late-stage lesions are treated by chemotherapy and radiation, which have changed little in 50 years, emphasizing the need for new treatment [1] . Characterization of the mechanism that promotes treatment resistance will provide novel treatment targets. Although the mechanism is unclear, pathways that promote DNA repair induce treatment resistance [3] , underscoring the importance of characterizing these proteins in SCCHN. Double-strand breaks (DSBs), the most dangerous type of DNA damage, are induced by radiation and chemotherapy [4] and DSBs are repaired primarily by homologous recombination (HR) or nonhomologous end joining (NHEJ) [3] . HR requires a DNA template, normally a homologous chromosome in germ cells or a sister chromatid in somatic cells. HR is essential for genetic diversity and transmission of genetic information between generations of cells and organisms. NHEJ occurs throughout the cell cycle and is required for physiologic processes including antigen receptor diversity and generation of antigen-specific antibodies [5] . NHEJ is usually inaccurate since DNA ends join without a template [6] . Error-prone or excessive repair promotes mutations, chromosome instability and cancer, whereas unrepaired DNA leads to cell death. In cancer, efficient repair of radiation- and chemotherapy-induced DSBs promotes treatment resistance with subsequent relapse. Therefore, inhibition of NHEJ would improve response to treatment. On the basis of meta-analyses of multiple SCCHN data sets, we nominated Thyroid hormone Receptor Interactor 13 (TRIP13 or HPV16E1BP) as an oncogene. TRIP13 is the mouse orthologue of pachytene checkpoint 2 (Pch2), a checkpoint for synapsis before DSB repair and recombination in yeast and Caenorhabditis elegans [7] , [8] . In mice, TRIP13 mediates DSB repair [9] , [10] ; however, the role of TRIP13 in humans has not been investigated. In this study, we investigated a mechanism by which TRIP13 promotes treatment resistance. Overexpression of TRIP13 in non-malignant cells leads to malignant transformation. High expression of TRIP13 in SCCHN promoted aggressive tumor growth, treatment resistance and enhanced repair of DNA damage. TRIP13-binding partners, including DNA-PKcs complex proteins mediating NHEJ, were identified using mass spectrometry. Repair-deficient reporter systems revealed that TRIP13 promotes NHEJ. Overexpression of TRIP13 sensitized SCCHN to an inhibitor of DNA-PKcs and impairment of TRIP13 ATPase activity diminishes its DSB repair efficiency. These findings define a mechanism of treatment resistance in SCCHN and emphasize the importance of targeting NHEJ to overcome treatment failure. TRIP13 is overexpressed in SCCHN Recent sequencing studies emphasized the limited number of mutations present in SCCHN [11] . Therefore, we performed meta-analysis of multiple SCCHN data sets ( Fig. 1a , left to right: Cromer Head-Neck, accession GSE2379 (ref. 12 ), Estilo Head-Neck, accession GSE13601 (ref. 13 ), Ye Head-Neck, accession GSE9844 (ref. 14 ), Kuriakose Head-Neck, accession GDS2520 (ref. 15 ), Ginos Head-Neck [16] , Toruner Head-Neck, accession GSE3524 (ref. 17 ), all available from Oncomine, Compendia Bioscience, Ann Arbor, MI, USA), to nominate potential novel oncogenes. TRIP13 was significantly upregulated in all six data sets interrogated ( Fig. 1a ). The Cancer Genome Atlas data set showed highly increased TRIP13 copy number (approximately four copies) in ~14% (40/290) of SCCHN patients ( Fig. 1b ). TRIP13 was nominated as an oncogene and is not mutated in SCCHN ( Supplementary Fig. 1A , left panel). TRIP13 copy number and gene expression frequency are increased in multiple cancers ( Supplementary Fig. 1A , middle and right panels). Compared with immortalized non-malignant keratinocytes, fluorescence in situ hybridization (FISH) showed increased TRIP13 copy number in SCCHN cells and tissue ( Fig. 1c , Supplementary Fig. 1B,C ). 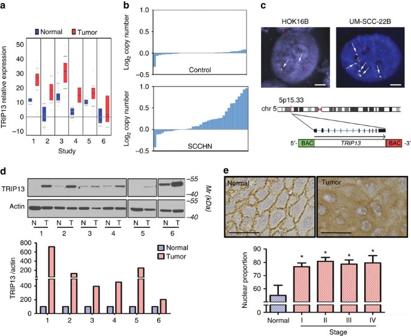Figure 1: TRIP13 is upregulated in SCCHN. (a) Meta-analysis showing TRIP13 upregulation in cancer compared with normal tissue. Left to right: Cromer-Head-Neck, Estilo-Head-Neck, Ye-Head-Neck, Kuriakose-Head-Neck, Ginos-Head-Neck, Toruner-Head-Neck (accession numbers are in Results section). (b) Analysis of 35 normal and 37 SCCHN cases showing TRIP13 DNA copy number increase in The Cancer Genome Atlas data set. (c) FISH detection ofTRIP13amplification in SCCHN cell line UM-SCC-22B compared with normal keratinocyte HOK16B. The 5′ (green) and 3′ (red) ends ofTRIP13were labelled. Colocalization of 5′ and 3′ ends (yellow) indicates a full copy ofTRIP13(white arrow; bar=2 μm). (d) Matched normal and tumour tissue lysates from SCCHN patients (n=18, 9 normal, 9 tumor) were immunoblotted with anti-TRIP13 and anti-actin antibodies. Signal intensity was quantified (arbitrary-densitometric-units, DU), normalized to actin and expressed and plotted as percent of its corresponding control (lower panel). (e) A TMA with SCCHN and normal tissue (n=72 cases, 12 normal, 60 SCCHN patients) was stained for TRIP13 with DAB detection (bar=30 μm). Staining proportion was scored and plotted (lower panel). Forward and stepwise variable selection procedures and the Likelihood Ration test were used for statistical analysis (P<0.05; * indicates statistically significant). Figure 1: TRIP13 is upregulated in SCCHN. ( a ) Meta-analysis showing TRIP13 upregulation in cancer compared with normal tissue. Left to right: Cromer-Head-Neck, Estilo-Head-Neck, Ye-Head-Neck, Kuriakose-Head-Neck, Ginos-Head-Neck, Toruner-Head-Neck (accession numbers are in Results section). ( b ) Analysis of 35 normal and 37 SCCHN cases showing TRIP13 DNA copy number increase in The Cancer Genome Atlas data set. ( c ) FISH detection of TRIP13 amplification in SCCHN cell line UM-SCC-22B compared with normal keratinocyte HOK16B. The 5′ (green) and 3′ (red) ends of TRIP13 were labelled. Colocalization of 5′ and 3′ ends (yellow) indicates a full copy of TRIP13 (white arrow; bar=2 μm). ( d ) Matched normal and tumour tissue lysates from SCCHN patients ( n =18, 9 normal, 9 tumor) were immunoblotted with anti-TRIP13 and anti-actin antibodies. Signal intensity was quantified (arbitrary-densitometric-units, DU), normalized to actin and expressed and plotted as percent of its corresponding control (lower panel). ( e ) A TMA with SCCHN and normal tissue ( n =72 cases, 12 normal, 60 SCCHN patients) was stained for TRIP13 with DAB detection (bar=30 μm). Staining proportion was scored and plotted (lower panel). Forward and stepwise variable selection procedures and the Likelihood Ration test were used for statistical analysis ( P <0.05; * indicates statistically significant). Full size image SCCHN exhibited high TRIP13 expression in tumor tissue compared with adjacent normal mucosa in paired normal and cancer tissue specimens ( Fig. 1d and bottom graph). In a tissue microarray (TMA), the intensity and proportion of TRIP13 were significantly higher in the nuclei in SCCHN compared with normal oral mucosa ( Fig. 1e , clinical data in Supplementary Table I). Together, these data indicate that TRIP13 is upregulated in SCCHN patients because of gene amplification. TRIP13 promotes proliferation invasion and cell survival TRIP13 mRNA and protein expression levels were verified using quantitative real-time PCR (Q-RT–PCR) ( Fig. 2a ) and immunoblot analysis ( Fig. 2b ) in SCCHN cell lines. In 10 of 12 SCCHN cell lines, TRIP13 was upregulated compared with non-malignant keratinocytes (HOK and HOK16B). 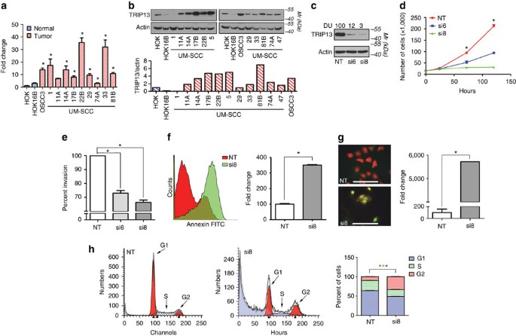Figure 2: Suppression of TRIP13 inhibits oncogenic phenotypes. (a) Total RNA from normal (HOK) and immortalized (HOK16B) keratinocytes and 10 SCCHN cell lines was used for Q-RT–PCR. Data were normalized to GAPDH and then to normal keratinocytes. (b) Lysates from SCCHN cell lines were immunoblotted with TRIP13 and actin. Signal intensity was quantified (DU), normalized to actin and plotted (lower panel). (c) UM-SCC-22B cells were transfected with two different siTRIP13 (si6, si8) or non-target siRNA (siNT). After 72 h cell lysates were immunoblotted with anti-TRIP13 and anti-actin. Signal intensity was normalized to actin and expressed as percent of control. (d) Cells were transfected with siTRIP13 or control NT siRNA and seeded and counted (days 1, 3 and 5) for proliferation assay. (e) Cells were transfected with siTRIP13 or control NT siRNA and seeded on matrigel-coated inserts. Invasion was quantified at 48 h post seeding. (f) Apoptosis was measured using flow cytometry and AnnexinV-FITC staining in cells transfected with siTRIP13-8 or control NT siRNA. (g) Cells transfected with siTRIP13-8 or siNT were seeded on coverslips. Apoptosis was visualized using the TUNEL Assay (green cells; bar=100 μm). (h) Cells, treated with siTRIP13-8 or siNT were synchronized and the distribution of cells in different phases of the cell cycle was determined using flow cytometry. Data represent three independent experiments performed in triplicate. Student’st-test with s.e.m.;P<0.02 (* indicates statistically significant). Figure 2: Suppression of TRIP13 inhibits oncogenic phenotypes. ( a ) Total RNA from normal (HOK) and immortalized (HOK16B) keratinocytes and 10 SCCHN cell lines was used for Q-RT–PCR. Data were normalized to GAPDH and then to normal keratinocytes. ( b ) Lysates from SCCHN cell lines were immunoblotted with TRIP13 and actin. Signal intensity was quantified (DU), normalized to actin and plotted (lower panel). ( c ) UM-SCC-22B cells were transfected with two different siTRIP13 (si6, si8) or non-target siRNA (siNT). After 72 h cell lysates were immunoblotted with anti-TRIP13 and anti-actin. Signal intensity was normalized to actin and expressed as percent of control. ( d ) Cells were transfected with siTRIP13 or control NT siRNA and seeded and counted (days 1, 3 and 5) for proliferation assay. ( e ) Cells were transfected with siTRIP13 or control NT siRNA and seeded on matrigel-coated inserts. Invasion was quantified at 48 h post seeding. ( f ) Apoptosis was measured using flow cytometry and AnnexinV-FITC staining in cells transfected with siTRIP13-8 or control NT siRNA. ( g ) Cells transfected with siTRIP13-8 or siNT were seeded on coverslips. Apoptosis was visualized using the TUNEL Assay (green cells; bar=100 μm). ( h ) Cells, treated with siTRIP13-8 or siNT were synchronized and the distribution of cells in different phases of the cell cycle was determined using flow cytometry. Data represent three independent experiments performed in triplicate. Student’s t -test with s.e.m. ; P <0.02 (* indicates statistically significant). Full size image Although expression data suggested that TRIP13 is overexpressed in SCCHN, the role of TRIP13 is unknown. Hence, we investigated the function of TRIP13 in SCCHN progression by performing proliferation, invasion and survival assays. In initial studies four different short interfering RNAs (siRNAs) against TRIP13 were evaluated ( Supplementary Fig. 1D,E ) in UM-SCC-22B and OSCC3, which have high endogenous TRIP13 ( Fig. 2b ). The siRNAs (si6, si8) showing the most sustained knockdown of TRIP13 ( Fig. 2c ) were used for proliferation and invasion studies. Downregulation of TRIP13 significantly decreased proliferation ( Fig. 2d ) and invasion ( Fig. 2e ). Similar findings were observed in OSCC3 ( Supplementary Fig. 2A through 2C) and UM-SCC-5 ( Supplementary Fig. 3A through 3C), two independent cell lines, which also overexpress TRIP13. si6 had a profound early effect on downregulation of TRIP13 ( Supplementary Fig. 1E ); however, downregulation was more sustained with si8 ( Fig. 2c ) across cell lines, likely because of apoptosis of cells transfected with si6. Hence, si8 was used for subsequent studies. To understand the impact of TRIP13 on cell survival, apoptosis was evaluated using flow cytometry in cells stained with FITC-Annexin V and propidium iodide (PI). Downregulation of TRIP13 significantly increased apoptosis in UM-SCC-22B ( Fig. 2f ), OSCC3 ( Supplementary Fig. 2D ) and UM-SCC-5 ( Supplementary Fig. 3D ). DNA fragmentation of apoptotic cells was visualized with fluorescein-labelled Brd-UTP (terminal deoxynucleotidyl transferase dUTP nick-end labeling, TUNEL) and quantified ( Fig. 2g , Supplementary Figs 2E and 3E ). To understand whether knockdown of TRIP13 has an impact on the cell cycle, SCCHN cells were synchronized, stained with PI and analysed using flow cytometry. Knockdown of TRIP13 led to fewer cells in the G1 and S phases and more in the G2 phase ( Fig. 2h , Supplementary Fig. 2F ). Cells arrested in G2 progress to apoptosis instead of moving into the M phase [18] . Together, these findings suggest that TRIP13 promotes oncogenic phenotypes in vitro . TRIP13 promotes tumour progression To investigate the function of TRIP13 in vivo , we attempted to generate SCCHN cell lines with stable downregulation of TRIP13. However, repeated attempts to generate these cells were unsuccessful, likely because of apoptosis. Using a different approach, we generated doxycycline-inducible shTRIP13- and control-SCCHN cell lines by transducing TRIPZ-shTRIP13 and shTRIPZ-control lentiviral particles in UM-SCC-22B and OSCC3. Mixed clonal populations were selected against puromycin. Knockdown was verified using immunoblot analysis ( Fig. 3a , Supplementary Fig. 4A , respectively) and proliferation ( Fig. 3b , Supplementary Fig. 4B ) assays. UM-SCC-22B-shTRIPZ-shTRIP13 (shTRIP13) and control (shControl) cells were injected subcutaneously in mice ( n =10). After 8 days (8d), similar-sized tumours appeared in both shcontrol and shTRIP13 groups and doxycycline administration was initiated ( n =5) in one and no-doxycycline was administered in the other groups ( n =5). The impact of doxycycline administration on tumour growth was rapid. Doxycycline-induced shTRIP13 significantly arrested tumour growth compared with doxycycline-treated control tumors ( Fig. 3c,d ). Tumour volume ( Fig. 3e ) and weight ( Fig. 3f ) were significantly less for doxycycline-induced shTRIP13. No significant difference in tumour size was observed in mice not administered doxycycline ( Supplementary Fig. 4C,D ). Proliferation and survival of tumour cells were investigated in these tumours; doxycycline-treated shTRIP13 tumours had significantly less mitoses ( Fig. 3g ), a marker of proliferation, and higher apoptosis ( Fig. 3h ), than corresponding control tumours. Furthermore, angiogenesis was quantified on tissue sections from chick chorioallantoic membrane (CAM) tumors generated from doxycycline-induced TRIP13 knockdown (TripZ) and control UM-SCC-22B cells. No significant difference in vessel length and number of junctions was observed ( Supplementary Fig. 4E ), suggesting that TRIP13 does not regulate angiogenesis. Together the in vitro and in vivo results support a tumorigenic role for TRIP13. 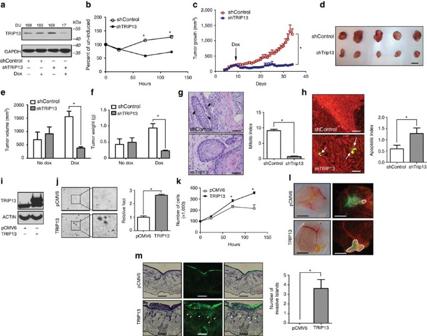Figure 3: TRIP13 is oncogenic. (a) UM-SCC-22B cells were stably transfected with inducible-shTRIP13 or shControl, and lysates from doxycycline-induced and non-induced cells were immunoblotted with TRIP13 and actin antibodies. Signal intensity was quantified, normalized to actin and expressed as percent of induced-shControl. (b) UM-SCC-22B-shControl and shTRIP13 cells were seeded, induced with 1 μg ml−1doxycycline and counted. Data represent three independent experiments performed in triplicate. Student’st-test with s.e.m.;P<0.03. (c) UM-SCC-22B-shControl and -shTRIP13 cells were injected subcutaneously into mice and induced with doxycycline after 8d. Tumours were measured daily for 34d. (d) Gross appearance of tumours; shControl (upper) and shTRIP13 (lower; bar=1 cm). Volume (e) and weight (f) of shControl and shTRIP13 tumors +/− doxycycline. (g) Mitoses/100 cells were quantified in five high-power fields on tumour sections from these mouse xenograft tumours (bar=60 μm). (h) A TUNEL assay on tumour sections was performed. Apoptotic cells (green)/100 cells in five high-power fields of each tumour were quantified (bar=25 μm). (i) NIH3T3 cells were transfected with pCMV6-Flag-TRIP13 or pCMV6-Flag. Cell lysates were immunoblotted with TRIP13 and actin antibodies. (j) NIH3T3-pCMV6 and NIH3T3-TRIP13 cells were cultured for 14d, stained with crystal violet and foci were counted (× 4 inset expanded). Data represent three independent experiments, each with three replicates. Student’st-test with s.e.m.;P<0.04. (k) NIH3T3-pCMV6 and NIH3T3-TRIP13 cells cultured in a 24-well plate were counted. Data represent one of three independent experiments, each with three replicates. Student’st-test with s.e.m.;P<0.03. (l) NIH3T3 cells stably expressing TRIP13 and pCMV6 were seeded on the CAM of a 10d-old chick embryo and grown for 3d. Gross appearance of the tumours is shown (bar=5 mm). (m) Haematoxylin–eosin staining (left) and green-fluorescent labelled cells (middle) and merged (right) panels show invasion of NIH3T3-TRIP13 cells (white arrow heads, bar=120 μm). The number of invasive islands was calculated from five representative fields. Student’st-test with s.e.m.;P<0.04 (* indicates statistically significant with correspondingP-values). Figure 3: TRIP13 is oncogenic. ( a ) UM-SCC-22B cells were stably transfected with inducible-shTRIP13 or shControl, and lysates from doxycycline-induced and non-induced cells were immunoblotted with TRIP13 and actin antibodies. Signal intensity was quantified, normalized to actin and expressed as percent of induced-shControl. ( b ) UM-SCC-22B-shControl and shTRIP13 cells were seeded, induced with 1 μg ml −1 doxycycline and counted. Data represent three independent experiments performed in triplicate. Student’s t -test with s.e.m. ; P <0.03. ( c ) UM-SCC-22B-shControl and -shTRIP13 cells were injected subcutaneously into mice and induced with doxycycline after 8d. Tumours were measured daily for 34d. ( d ) Gross appearance of tumours; shControl (upper) and shTRIP13 (lower; bar=1 cm). Volume ( e ) and weight ( f ) of shControl and shTRIP13 tumors +/− doxycycline. ( g ) Mitoses/100 cells were quantified in five high-power fields on tumour sections from these mouse xenograft tumours (bar=60 μm). ( h ) A TUNEL assay on tumour sections was performed. Apoptotic cells (green)/100 cells in five high-power fields of each tumour were quantified (bar=25 μm). ( i ) NIH3T3 cells were transfected with pCMV6-Flag-TRIP13 or pCMV6-Flag. Cell lysates were immunoblotted with TRIP13 and actin antibodies. ( j ) NIH3T3-pCMV6 and NIH3T3-TRIP13 cells were cultured for 14d, stained with crystal violet and foci were counted (× 4 inset expanded). Data represent three independent experiments, each with three replicates. Student’s t -test with s.e.m. ; P <0.04. ( k ) NIH3T3-pCMV6 and NIH3T3-TRIP13 cells cultured in a 24-well plate were counted. Data represent one of three independent experiments, each with three replicates. Student’s t -test with s.e.m. ; P <0.03. ( l ) NIH3T3 cells stably expressing TRIP13 and pCMV6 were seeded on the CAM of a 10d-old chick embryo and grown for 3d. Gross appearance of the tumours is shown (bar=5 mm). ( m ) Haematoxylin–eosin staining (left) and green-fluorescent labelled cells (middle) and merged (right) panels show invasion of NIH3T3-TRIP13 cells (white arrow heads, bar=120 μm). The number of invasive islands was calculated from five representative fields. Student’s t -test with s.e.m. ; P <0.04 (* indicates statistically significant with corresponding P -values). Full size image To establish an oncogenic role, we interrogated whether TRIP13 could transform non-malignant cells using the focus formation (transformation) assay in NIH3T3 fibroblasts. NIH3T3 cells grow to confluence and senesce since contact inhibition prevents cell stratification [19] . However, overexpression of TRIP13 in NIH3T3 cells ( Fig. 3i ) led to significantly more cellular stratification, that is, focus formation ( Fig. 3j ), and proliferation ( Fig. 3k ) than control NIH3T3-pCMV6 cells. To conclusively establish the oncogenicity of TRIP13, tumour growth of NIH3T3-TRIP13 cells was verified in vivo using the CAM assay. After 3d, green fluorescent protein (GFP)-labelled NIH3T3-TRIP13 cells formed a three-dimensional (3D) tumour ( Fig. 3l ; n =5; broken lines) in contrast to the thin layer of control cells. NIH3T3-TRIP13 cells invaded the underlying mesenchymal tissue ( Fig. 3m , lower panel, arrowheads and graph) in contrast to control (NIH3T3-pCMV6) cells, which remained as a single layer on the surface of the CAM ( Fig. 3m , upper panel and graph). In a complementary approach, TRIP13 was stably overexpressed in UM-SCC-1, a cell line with low endogenous TRIP13 ( Fig. 2b ). Overexpression was verified using immunoblot analysis ( Fig. 4a ). UM-SCC-1-TRIP13 cells exhibited significantly higher proliferation ( Fig. 4b ), invasion ( Fig. 4c ) and migration ( Fig. 4d ) compared with control (UM-SCC-1-pCMV6) cells. To investigate the in vivo impact of overexpression of TRIP13, cells were injected subcutaneously in mice ( n =10) and tumours were grown until mice became moribund. Control tumours (UM-SCC-1-pCMV6; Fig. 4e , pCMV6, n =5) grew significantly slower than TRIP13-overexpressing tumours (UM-SCC-1-TRIP13; Fig. 4f , TRIP13, n =5). Moreover, mice with TRIP13 tumours had poorer survival than those with control tumours ( Fig. 4g ; P =0.0019, log-rank). This correlated with significantly increased tumour size ( Fig. 4h ). Tissue sections and immunohistochemical staining were used to determine the mitotic index and proliferating cell nuclear antigen-positive cells, respectively, both measures of proliferative activity. UM-SCC-1-TRIP13 tumours had significantly more mitoses ( Fig. 4i ), a higher proliferative index ( Fig. 4j ) and a lower apoptotic index ( Fig. 4k ) than control tumours, consistent with our in vitro findings that TRIP13 promotes survival. Together, the in vitro and in vivo studies establish TRIP13 as an oncogene. 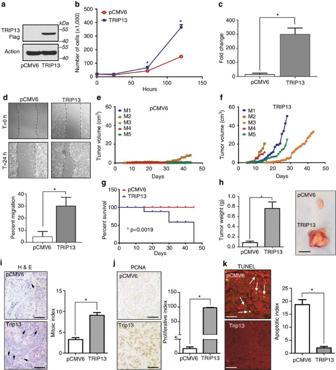Figure 4: TRIP13 promotes tumour growth. UM-SCC-1 cells were stably transfected with pCMV6-Flag and pCMV6-Flag-TRIP13. (a) Cell lysates were immunoblotted with anti-Flag and anti-actin antibodies. (b) UM-SCC-1-pCMV6 and UM-SCC-1-TRIP13 cells were seeded and counted for proliferation. Data represent three independent experiments with three replicates in each experiment. (Student’st-test with s.e.m.;P<0.002). (c) UM-SCC-1-pCMV6 and UM-SCC-1-TRIP13 cells were seeded on matrigel-coated inserts and invasion was quantified 48 h later. Data represent three independent experiments with three replicates in each experiment. (Student’st-test with s.e.m.;P<0.002). (d) Cells were seeded at ~95% confluence and treated with mitomycin-C. After 24 h, a scratch was performed and the migration distance was quantified (bottom panel). (e) Stable UM-SCC-1-pCMV6 and (f) UM-SCC-1-TRIP13 cells were injected subcutaneously in mice (n=5 in each group). Tumours were measured daily till mice were moribund. Tumour volume was calculated. (g) Survival curves for mice injected with UM-SCC-1-pCMV6 or UM-SCC-1-TRIP13 were plotted. (h) Tumour weight (left) and a representative xenograft tumour from UM-SCC-1-pCMV6 and UM-SCC-1-TRIP13 (right) are shown (bar=1 cm). (i) Haematoxylin–eosin staining of xenograft tumours and the mitotic index calculated from the average of all tumours (bar=60 μm;n=10, 5 in each group). (j) Immunohistochemical staining of the xenograft tumors with proliferating cell nuclear antigen. Proliferative index represents the average staining in 100 cells in each of the tumours (bar=60 μm). (k) TUNEL staining was performed for detecting apoptotic cells. Apoptotic index represents the average number of apoptotic cells per s100 cells in each of the tumours (bar=100 μm). Student’st-test with s.e.m.;P<0.05 (* indicate statistically significant with correspondingP-values). Figure 4: TRIP13 promotes tumour growth. UM-SCC-1 cells were stably transfected with pCMV6-Flag and pCMV6-Flag-TRIP13. ( a ) Cell lysates were immunoblotted with anti-Flag and anti-actin antibodies. ( b ) UM-SCC-1-pCMV6 and UM-SCC-1-TRIP13 cells were seeded and counted for proliferation. Data represent three independent experiments with three replicates in each experiment. (Student’s t -test with s.e.m. ; P <0.002). ( c ) UM-SCC-1-pCMV6 and UM-SCC-1-TRIP13 cells were seeded on matrigel-coated inserts and invasion was quantified 48 h later. Data represent three independent experiments with three replicates in each experiment. (Student’s t -test with s.e.m. ; P <0.002). ( d ) Cells were seeded at ~95% confluence and treated with mitomycin-C. After 24 h, a scratch was performed and the migration distance was quantified (bottom panel). ( e ) Stable UM-SCC-1-pCMV6 and ( f ) UM-SCC-1-TRIP13 cells were injected subcutaneously in mice ( n =5 in each group). Tumours were measured daily till mice were moribund. Tumour volume was calculated. ( g ) Survival curves for mice injected with UM-SCC-1-pCMV6 or UM-SCC-1-TRIP13 were plotted. ( h ) Tumour weight (left) and a representative xenograft tumour from UM-SCC-1-pCMV6 and UM-SCC-1-TRIP13 (right) are shown (bar=1 cm). ( i ) Haematoxylin–eosin staining of xenograft tumours and the mitotic index calculated from the average of all tumours (bar=60 μm; n =10, 5 in each group). ( j ) Immunohistochemical staining of the xenograft tumors with proliferating cell nuclear antigen. Proliferative index represents the average staining in 100 cells in each of the tumours (bar=60 μm). ( k ) TUNEL staining was performed for detecting apoptotic cells. Apoptotic index represents the average number of apoptotic cells per s100 cells in each of the tumours (bar=100 μm). Student’s t -test with s.e.m. ; P <0.05 (* indicate statistically significant with corresponding P -values). Full size image TRIP13 mediates treatment resistance Given the role of TRIP13 in promoting cell survival, we investigated its effects in response to cisplatin (CDDP) chemotherapy and ionizing radiation (IR)-induced cell death. In initial studies, the IC 50 for CDDP in UM-SCC-22B and OSCC3 were determined to be 5 and 2 μM, respectively ( Supplementary Fig. 4F,G , respectively). UM-SCC-22B ( Fig. 5a ) and OSCC3 ( Supplementary Fig. 5A ) cells with downregulated TRIP13 were treated with CDDP and cell number was counted. Cells treated with siTRIP13+CDDP grew significantly slower than control siNT+CDDP, suggesting a role for TRIP13 in chemoresistance. The inhibitory effect of siTRIP13 was greater than that of CDDP; combination treatment (siTRIP13+CDDP) had an additive effect. Clonogenic assays showed that survival of siTRIP13+IR cells was significantly less than control NT+IR cells ( Fig. 5b , Supplementary Fig. 5B ), consistent with a role for TRIP13 in promoting IR resistance. DNA fragmentation, a marker of apoptosis, was greater in siTRIP13+IR than in control NT+IR cells ( Fig. 5c , Supplementary Fig. 5C ). 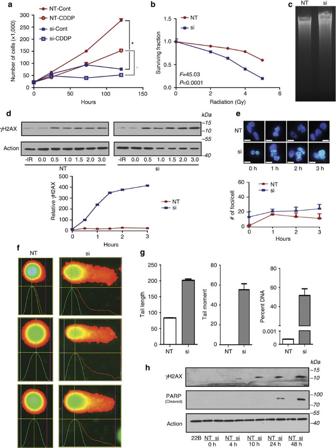Figure 5: Suppression of TRIP13 increases DNA damage. UM-SCC-22B cells were transfected with siTRIP13 or siNT. (a) Cells were treated with 5 μM CDDP for 2 h and counted 1d, 3d and 5d post treatment. Data represent three independent experiments with three replicates in each experiment. Student’st-test with s.e.m.;P<0.04. (b) Cells transfected with siNT or siTRIP13 were seeded at siNT (3,000) and siTRIP13 (30,000) and 5d post seeding, cells were irradiated (2, 3, 4 and 5 Gy), then grown for 10d. Crystal violet-stained colonies were counted. Data represent three independent experiments with three replicates in each experiment. (c) Cells were synchronized with nocodozole and irradiated (4 Gy). Genomic DNA was isolated, electrophoresed and visualized with ethidium bromide. (d) Cells were irradiated (4 Gy) and lysates were collected at 30, 60 and 90, and 2, 3 and 4 h. Lysates were immunoblotted with anti-γH2 AX and anti-actin antibodies. Signal intensity was quantified and plotted over time (bottom graph). (e) Immunofluorescence with anti-γH2AX (green) and DAPI nuclear counterstain was performed after cells were irradiated (4 Gy). The average number of γH2AX foci per cell was calculated for NT and siTRIP13 and plotted over time (bottom graph; bar=20 μm). (f) Comet assay of cells transfected with siNT and siTRIP13 showing DNA damage (three fields shown). (g) Tail length, moment and percent DNA in the tail were calculated. (h) Time course of γH2 AX and PARP cleavage were assessed with lysates prepared from UM-SCC-22B cells transfected with siNT and siTRIP13 and immunoblotted with anti-γH2AX, anti-cleaved-PARP and anti-actin antibodies (* indicates statistically significant). Figure 5: Suppression of TRIP13 increases DNA damage. UM-SCC-22B cells were transfected with siTRIP13 or siNT. ( a ) Cells were treated with 5 μM CDDP for 2 h and counted 1d, 3d and 5d post treatment. Data represent three independent experiments with three replicates in each experiment. Student’s t -test with s.e.m. ; P <0.04. ( b ) Cells transfected with siNT or siTRIP13 were seeded at siNT (3,000) and siTRIP13 (30,000) and 5d post seeding, cells were irradiated (2, 3, 4 and 5 Gy), then grown for 10d. Crystal violet-stained colonies were counted. Data represent three independent experiments with three replicates in each experiment. ( c ) Cells were synchronized with nocodozole and irradiated (4 Gy). Genomic DNA was isolated, electrophoresed and visualized with ethidium bromide. ( d ) Cells were irradiated (4 Gy) and lysates were collected at 30, 60 and 90, and 2, 3 and 4 h. Lysates were immunoblotted with anti-γH2 AX and anti-actin antibodies. Signal intensity was quantified and plotted over time (bottom graph). ( e ) Immunofluorescence with anti-γH2AX (green) and DAPI nuclear counterstain was performed after cells were irradiated (4 Gy). The average number of γH2AX foci per cell was calculated for NT and siTRIP13 and plotted over time (bottom graph; bar=20 μm). ( f ) Comet assay of cells transfected with siNT and siTRIP13 showing DNA damage (three fields shown). ( g ) Tail length, moment and percent DNA in the tail were calculated. ( h ) Time course of γH2 AX and PARP cleavage were assessed with lysates prepared from UM-SCC-22B cells transfected with siNT and siTRIP13 and immunoblotted with anti-γH2AX, anti-cleaved-PARP and anti-actin antibodies (* indicates statistically significant). Full size image IR and CDDP promote apoptosis by inducing DSB, the most lethal form of DNA damage [4] . Therefore, we investigated the effects of TRIP13 on DSB repair. Since histone H2AX is phosphorylated at Ser-139 (γH2AX) in response to DSBs [20] , γH2AX expression was used to quantify DSBs. Loss of γH2AX indicates efficient DSB repair, whereas persistent γH2AX indicates impaired DSB repair [21] . In irradiated UM-SCC-22B and OSCC3, knockdown of TRIP13 correlated with γH2AX accumulation ( Fig. 5d , Supplementary Fig. 5D , respectively). Spontaneous DSBs and DNA repair occur during cell proliferation. Therefore, we investigated DSBs in cells transfected with NT and siTRIP13 and observed significantly more γH2AX foci/cell in siTRIP13 than NT cells ( Fig. 5e , Supplementary Fig. 5E ). These studies suggest that loss of TRIP13 promotes accumulation of DNA damage. Hence, we evaluated the impact of TRIP13 on DSB by the comet assay in NT and siTRIP13 cells ( Fig. 5f , Supplementary Fig. 5F ). Cells with siTRIP13 showed significantly increased DNA damage in UM-SCC-22B ( Fig. 5g ) and OSCC3 ( Supplementary Fig. 5G ). To determine whether siTRIP13-mediated DSB induces apoptosis or apoptosis induces DSB, we performed a time course experiment to investigate the sequence between γH2AX and apoptosis after knockdown of TRIP13 ( Fig. 5h ). We observed that γH2AX (marker of DSBs) precedes PARP cleavage (marker of apoptosis). γH2AX was observed in siTRIP13 cells as early as 4 h post transfection, whereas cleaved PARP appeared at 24 h post transfection indicating siTRIP13-mediated DSB precedes apoptosis ( Fig. 5h ). Taken together, these studies support that TRIP13 promotes treatment resistance via enhanced DNA repair. TRIP13 has an ATPase domain, a hallmark of AAA-ATPase proteins [22] that mediate protein–DNA or protein–protein complex assembly [23] . To identify proteins that interact with TRIP13, we performed LC-tandem mass spectrometry [24] . Flag-tagged TRIP13 was purified with Sigma-Flag-Beads (M2) from UM-SCC-1 cells stably overexpressing FLAG-TRIP13, stained and immunoblotted ( Supplementary Fig. 6A ). Interacting proteins were identified using the X!Tandem/Trans-Proteomic Pipeline software [25] . Proteins with a Protein Prophet probability score >0.9 (error rate <2%) were considered to be positive identifications and functionally classified ( Supplementary Table 2 ). These proteins were entered in the string database ( http://string-db.org/ ) to predict the interaction network. Molecules out of the network were deleted and an interaction map consisting of 18 molecules is summarized ( Fig. 6a ). The greatest interaction network concepts determined from the KEGG pathway analysis were NHEJ and Cell cycle/DNA repair pathways ( Supplementary Table 3 ). NHEJ/DNA repair group proteins included KU70 (XRCC6), KU80 (XRCC5) and DNA-PKcs (PRKDC; Fig. 6a ). Mass spectrometry sequence coverage of these interacting proteins is shown ( Fig. 6b ). The interactions were further validated using immunoprecipitation with TRIP13 antibody in UM-SCC-22B ( Fig. 6c ) and OSCC3 ( Supplementary Fig. 6B ). KU70, KU80 and DNA-PKcs co-immunoprecipitated with TRIP13 but not control IgG ( Fig. 6c , Supplementary Fig. 6B ). To verify that TRIP13 interacted with each protein directly, not via DNA, immunoprecipitation was also performed in the presence of ethidium bromide. In a complementary experiment, KU70, KU80 and DNA-PKcs were immunoprecipitated with corresponding antibodies and immunoblotted with TRIP13 antibody. TRIP13 co-immunoprecipitated with each of these proteins but not with control IgG ( Fig. 6d , Supplementary Fig. 6C ), confirming interaction with DNA-repair proteins in SCCHN. 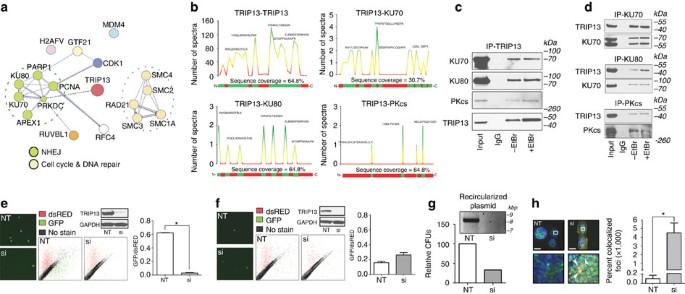Figure 6: TRIP13 promotes NHEJ. (a) Flag-tagged TRIP13 was purified from stable UM-SCC-1-TRIP13 and analysed using mass spectrometry for TRIP13-binding proteins. An enrichment network, derived from string database of TRIP13 interactors that links NHEJ proteins as well as chromosomal integration and repair signatures. (b) Peptide coverage for TRIP13 and TRIP13-interacting proteins for the NHEJ pathway are shown. (c) TRIP13 was immunoprecipitated in the presence or absence of ethidium bromide and immunoblotted with anti-KU70, KU80, DNA-PKcs and TRIP13 antibodies. (d) KU70, KU80 and DNA-PKcs were immunoprecipitated in the presence or absence of ethidium bromide with respective antibodies and immunoblotted with IP antibodies and anti-TRIP13 antibody. (e) HCC1937 cells stably expressing NHEJ (e) and HR (f) reporter constructs were transfected with siTRIP13 or NT. Forty-eight hours later, these cells were co-transfected with dsRed and I-Sce-1 plasmids. NHEJ and HR were quantified by GFP and dsRed expression using flow cytometry and quantified (right panel). (g) Mini-NHEJ extract from UM-SCC-22B cells transfected with NT or siTRIP13 was incubated with linearized plasmid with non-cohesive ends. The end joining product (recircularized plasmid) was purified, electrophoresed and visualized with ethidium bromide. Bacteria were transformed with recircularized plasmid and colonies were counted (bottom graph). (h) UM-SCC-22B-NT or -siTRIP13 cells were stained with γH2AX (green) and Rad51 (red) antibodies and DAPI (blue; bar=20 μm). Rad51/γH2AX colocalized foci (orange; × 5 inset expanded) were quantified (right graph). Student'st-test with s.e.m.P<0.02, * indicates statistically significant. Figure 6: TRIP13 promotes NHEJ. ( a ) Flag-tagged TRIP13 was purified from stable UM-SCC-1-TRIP13 and analysed using mass spectrometry for TRIP13-binding proteins. An enrichment network, derived from string database of TRIP13 interactors that links NHEJ proteins as well as chromosomal integration and repair signatures. ( b ) Peptide coverage for TRIP13 and TRIP13-interacting proteins for the NHEJ pathway are shown. ( c ) TRIP13 was immunoprecipitated in the presence or absence of ethidium bromide and immunoblotted with anti-KU70, KU80, DNA-PKcs and TRIP13 antibodies. ( d ) KU70, KU80 and DNA-PKcs were immunoprecipitated in the presence or absence of ethidium bromide with respective antibodies and immunoblotted with IP antibodies and anti-TRIP13 antibody. ( e ) HCC1937 cells stably expressing NHEJ ( e ) and HR ( f ) reporter constructs were transfected with siTRIP13 or NT. Forty-eight hours later, these cells were co-transfected with dsRed and I-Sce-1 plasmids. NHEJ and HR were quantified by GFP and dsRed expression using flow cytometry and quantified (right panel). ( g ) Mini-NHEJ extract from UM-SCC-22B cells transfected with NT or siTRIP13 was incubated with linearized plasmid with non-cohesive ends. The end joining product (recircularized plasmid) was purified, electrophoresed and visualized with ethidium bromide. Bacteria were transformed with recircularized plasmid and colonies were counted (bottom graph). ( h ) UM-SCC-22B-NT or -siTRIP13 cells were stained with γH2AX (green) and Rad51 (red) antibodies and DAPI (blue; bar=20 μm). Rad51/γH2AX colocalized foci (orange; × 5 inset expanded) were quantified (right graph). Student's t -test with s.e.m. P <0.02, * indicates statistically significant. Full size image DSBs are primarily repaired by accurate HR or error-prone NHEJ. Since KU70, KU80 and DNA-PKcs are members of the NHEJ repair complex [4] , we investigated the involvement of TRIP13 in NHEJ using reporter constructs [26] in the host cell reactivation system of HCC1937, a BRCA1 mutant cell line. The absence of BRCA1 in these cells inhibits HR, leaving NHEJ as the default repair pathway. HCC1937 cells stably transfected with NHEJ ( Fig. 6e ) or HR ( Fig. 6f ) reporter constructs were transiently transfected with NT or siTRIP13. Forty-eight hours later, the cells were co-transfected with the rare cutting endonuclease I-SceI expression plasmid and a transfection efficiency control plasmid (pDsRed2-N1), and 72 h later were analysed using flow cytometry. The I-SceI endonuclease induces DSBs in the reporter GFP cassette (schematics in Supplementary Fig. 6D,E ). When the two ends of the DSB are joined by NHEJ or HR, GFP is expressed. The relative efficiency of DSB repair was calculated as the ratio of GFP+/DsRed+ cells. GFP expression was significantly decreased in HCC1937-NHEJ-siTRIP13 compared with HCC1937-NHEJ-siNT ( Fig. 6e ), consistent with a role for TRIP13 in NHEJ. As a negative control for these HR-deficient cells, siTRIP13 had minimal impact on HR reporter expression ( Fig. 6f ). To verify that TRIP13 facilitates NHEJ, a mini-NHEJ assay was performed with linearized plasmid with non-cohesive ends. In this assay (See Supplementary Fig. 7a ), recircularization of linearized plasmid occurs via NHEJ because of the absence of DNA template necessary for HR. Mini-NHEJ extracts from UM-SCC-22B and OSCC3 with siTRIP13 or siNT were incubated with linearized plasmid and recircularization was evaluated on agarose gels ( Fig. 6g , Supplementary Fig. 6F , respectively) followed by transformation into competent bacteria and colony counting. When incubated with extracts from siTRIP13 cells, recircularized plasmid was undetectable and the number of colonies was reduced compared with siNT ( Fig. 6g , Supplementary Fig. 6F ). Recircularization of plasmid DNA was confirmed by generating PCR product from the primers P1-Forward and Reverse ( Supplementary Table 4 ; Supplementary Fig. 7A,B ) and sequence confirmation of base loss in NHEJ ( Supplementary Fig. 7C ). Moreover a semiquantitative PCR of 15 cycles showed reduced rejoined products when the rejoining reaction was performed with siTRIP13- versus NT extracts from three SCCHN cell lines ( Supplementary Fig. 7D ). Together, these findings show that TRIP13 is involved in the NHEJ pathway. HR pathway protein RAD51 translocates from the cytoplasm to the nucleus to accumulate at DSBs. To investigate the involvement of TRIP13 in HR, γH2Ax/Rad51 colocalization foci were quantified in UM-SCC-22B. TRIP13 expression was inversely correlated with γH2AX/Rad51 colocalization ( Fig. 6h ), suggesting that in HR-competent cells, DSB repair defaults to the HR pathway when TRIP13 is downregulated. Similar results were obtained with OSCC3 ( Supplementary Fig. 8A ). Together, our findings show that TRIP13 promotes NHEJ in HR-competent cells and that HR occurs when TRIP13 is downregulated. Induction of the NHEJ pathway confers treatment resistance making DNA-PKcs an attractive target in clinical trials [27] . After establishing that overexpression of TRIP13 drives treatment resistance via NHEJ, we hypothesized that SCCHN cells overexpressing TRIP13 would be more sensitive to a DNA-PKcs inhibitor than cells with low expression of TRIP13. To investigate this possibility, UM-SCC-1-pCMV6 and UM-SCC-1-TRIP13 cells were treated with multiple concentrations of NU7026 (100 nM to 10 μM, Supplementary Fig. 8B,C ), a DNA-PKcs inhibitor. Autophosphorylation of DNA-PKcs at Ser 2056 and proliferation were assessed. Control cells were less sensitive to NU7026 with respect to inhibition of DNA-PKcs’ phosphorylation and proliferation ( Supplementary Fig. 8B,C , left panels, respectively) than TRIP13-overexpressing cells ( Supplementary Fig. 8B,C , right panels, respectively). Furthermore, cells overexpressing TRIP13 (UM-SCC-1-TRIP13) were more sensitive to NU7026, with an IC 50 of 10 μM compared with 13 μM for control cells ( Fig. 7a ). To determine the effects on proliferation, UM-SCC-1-TRIP13 and UM-SCC-1-pCMV6 cells were treated with NU7026 ( Fig. 7b ). Using a mixed-effects model to account for correlation among repeat measurements, we observed the difference in the mean slope over time with and without NU7026 in Control- versus TRIP13-overexpressing groups. Importantly, the differences in slopes for the TRIP13 group (±NU7026) were significantly larger than the differences between control-pCMV6 cells ( Fig. 7b ), confirming that high expression of TRIP13 increases sensitivity to the NHEJ inhibitor. In addition, when NHEJ is blocked with NU7026, Rad51/γH2AX foci increased significantly ( Fig. 7c ). Importantly, similar results were observed in vivo . In the CAM, NU7026-mediated inhibition of tumour growth and metastasis was greater with TRIP13 than control cells. UM-SCC-1-pCMV6 cells±NU7026 exhibited no significant difference in tumour size ( Fig. 7d ), whereas NU7026 significantly inhibited growth of UM-SCC-1-TRIP13 tumours ( Fig. 7e ). More importantly, metastasis of these cells to the lower CAM, as detected using fluorescence microscopy ( Fig. 7f , left panel) and quantitative ALU-PCR for Lower CAM and liver [28] ( Fig. 7f , right top and bottom panels, respectively), was inhibited by NU7026. Together, these data show that TRIP13 promotes DSB repair and treatment resistance via the NHEJ pathway. Importantly, by favouring NHEJ, TRIP13 inhibits the intact HR pathway in SCCHN. 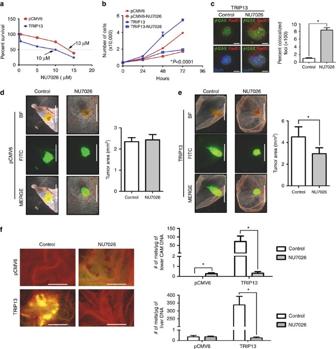Figure 7: TRIP13 overexpression is sensitized to NHEJ protein DNA-PKcs. (a) The IC50for NU7026 in UM-SCC-1-pCMV6 (13 μM) and -TRIP13 (10 μM) cells were determined. (b) UM-SCC-1-pCMV6 or -TRIP13 cells were seeded and 24 h later were treated with 10 μM NU7026 and subsequently cells were counted on 24, 48 and 72 h post NU7026 treatment. (Student’st-test with s.e.m.;P<0.0001). (c) UM-SCC-1-pCMV6 or -TRIP13 treated with 10 μM NU7026 for 72 h stained for γH2AX (green), Rad51 (red) and DAPI (blue; bar=20 μm). Colocalized foci (γH2AX/Rad51, orange) were quantified. Student’st-test with s.e.m.;P<0.003. (d,e) UM-SCC-1-pCMV6 (d) and UM-SCC-1-TRIP13 (e) cells (1 × 106) were labelled with green Cell-tracker and seeded on the CAM of a 10d-old chick embryo. Twenty-four hours later, 200 μM Nu7026 was added on top of the developing tumour. After 8d, the upper CAM was harvested, fixed and photographed (brightfield and GFP) and merged (bar=5 mm). Tumour size was quantified (corresponding right graph;d,e). Student’st-test with s.e.m.;P<0.05. (f) Metastasis to the lower CAM was evaluated by fluorescently labelled cells (left panel, bar=2 mm) and metastasis in lower CAM and liver was determined by quantitative-Alu-PCR (right top and bottom panels, respectively). Student’st-test with s.e.m.;P<0.001. Data are representative of two independent experiments, five replicates in each group (* indicates statistically significant with correspondingP-values). Figure 7: TRIP13 overexpression is sensitized to NHEJ protein DNA-PKcs. ( a ) The IC 50 for NU7026 in UM-SCC-1-pCMV6 (13 μM) and -TRIP13 (10 μM) cells were determined. ( b ) UM-SCC-1-pCMV6 or -TRIP13 cells were seeded and 24 h later were treated with 10 μM NU7026 and subsequently cells were counted on 24, 48 and 72 h post NU7026 treatment. (Student’s t -test with s.e.m. ; P <0.0001). ( c ) UM-SCC-1-pCMV6 or -TRIP13 treated with 10 μM NU7026 for 72 h stained for γH2AX (green), Rad51 (red) and DAPI (blue; bar=20 μm). Colocalized foci (γH2AX/Rad51, orange) were quantified. Student’s t -test with s.e.m. ; P <0.003. ( d , e ) UM-SCC-1-pCMV6 ( d ) and UM-SCC-1-TRIP13 ( e ) cells (1 × 10 6 ) were labelled with green Cell-tracker and seeded on the CAM of a 10d-old chick embryo. Twenty-four hours later, 200 μM Nu7026 was added on top of the developing tumour. After 8d, the upper CAM was harvested, fixed and photographed (brightfield and GFP) and merged (bar=5 mm). Tumour size was quantified (corresponding right graph; d , e ). Student’s t -test with s.e.m. ; P <0.05. ( f ) Metastasis to the lower CAM was evaluated by fluorescently labelled cells (left panel, bar=2 mm) and metastasis in lower CAM and liver was determined by quantitative-Alu-PCR (right top and bottom panels, respectively). Student’s t -test with s.e.m. ; P <0.001. Data are representative of two independent experiments, five replicates in each group (* indicates statistically significant with corresponding P -values). Full size image TRIP13 has an ATPase domain, a hallmark of AAA-ATPase proteins [22] that mediate protein–DNA or protein–protein complex assembly [23] . To determine whether the ATPase activity mediates the oncogenic activity of TRIP13, we generated TRIP13 mutants by altering amino acids at the conserved Walker A motif with site-directed mutagenesis or by deleting the conserved ATPase domain ( Fig. 8a ). The Walker A motif is required for ATP-binding activity [29] . The ATPase domain is required for diverse activities of AAA-ATPase proteins [30] . Expression of TRIP13 mt (TRIP13 G184A ) and TRIP13 Δmt (TRIP13 Δ293–312 ) mutant proteins was verified after transient transfection in COS-1 ( Fig. 8b ). ATPase enzymatic activity, assessed using the malachite green ATPase assay, was deficient with both mutant constructs when compared with wild-type TRIP13 ( Fig. 8c ). The deficiency of the ATPase activity also impaired proliferative activity ( Fig. 8d ). Similar findings were observed in UM-SCC-1 ( Fig. 8e–g ). Moreover, in TRIP13-overexpressing cells the low γH2AX is consistent with more efficient DSB repair compared to control pCMV6 cells ( Fig. 8h lane 2 compared with lane 1). TRIP13-mediated repair was impaired when the ATPase domain was mutated ( Fig. 8h lanes 3 and 4 compared with lane 2). The loss of ATPase activity also impaired TRIP13-mediated tumour growth on the CAM ( Fig. 8i,j ). 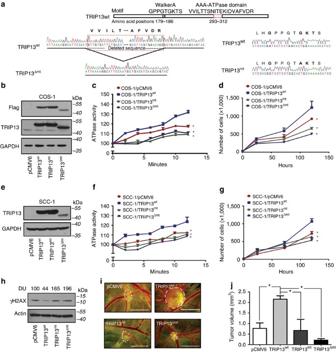Figure 8: Mutation of the conserved domain of TRIP13 impairs tumorigenesis. (a) Schematic presentation of conserved sequence motif of wild-type TRIP13 (TRIP13wt). The deleted and site-directed mutagenesis sites used for generation of TRIP13 mutants are shown. (b) Expression of Flag-tagged TRIP13 mutants was verified in COS-1 cells transiently overexpressing mutant proteins with antibodies to anti-Flag, anti-TRIP13 and anti-GAPDH antibodies. (c) A malachite green ATPase activity assay was performed with TRIP13 mutant proteins as well as with wild-type TRIP13 and pCMV6 control. ATPase activity was measured and normalized for 1 μg of each protein and was finally expressed as percent of corresponding activity at 0-min time point and graphed. Student’st-test with s.e.m.;P<0.04. (d) Proliferation assay was performed with COS-1 cells transiently overexpressing TRIP13 mutants. Student’st-test with s.e.m.;P<0.02. (e) Expression of mutant or wild-type Flag-tagged TRIP13 in stably expressing UM-SCC-1 cells was verified with anti-TRIP13 and anti-GAPDH antibodies. (f) A malachite green ATPase activity assay was performed with these cells. Student’st-test with s.e.m.;P<0.05. (g) A proliferation assay was performed with UM-SCC-1 cells stably overexpressing mutant or wild-type TRIP13 proteins along with control pCMV6 empty vector. Student’st-test with s.e.m.;P<0.04. (h) UM-SCC-1 cells stably expressing wild-type or mutant TRIP13 or control cells (pCMV6) were immunoblotted with anti-γH2AX, anti-actin antibodies and quantified (DU). (i) Mixed clonal population of UM-SCC-1 cells stably expressing wild-type or mutant TRIP13 or control cells were placed (1 × 106cells each) on the CAM (n=20, 5 in each group: two independent experiments). After incubating for 7 days, the upper CAM was excised and photographed (bar=5 mm). (j) The tumours (dotted boundary line) were measured and tumour volume was calculated. Student’st-test with s.e.m.;P<0.01 (* indicates statistically significant with correspondingPvalues). Figure 8: Mutation of the conserved domain of TRIP13 impairs tumorigenesis. ( a ) Schematic presentation of conserved sequence motif of wild-type TRIP13 (TRIP13 wt ). The deleted and site-directed mutagenesis sites used for generation of TRIP13 mutants are shown. ( b ) Expression of Flag-tagged TRIP13 mutants was verified in COS-1 cells transiently overexpressing mutant proteins with antibodies to anti-Flag, anti-TRIP13 and anti-GAPDH antibodies. ( c ) A malachite green ATPase activity assay was performed with TRIP13 mutant proteins as well as with wild-type TRIP13 and pCMV6 control. ATPase activity was measured and normalized for 1 μg of each protein and was finally expressed as percent of corresponding activity at 0-min time point and graphed. Student’s t -test with s.e.m. ; P <0.04. ( d ) Proliferation assay was performed with COS-1 cells transiently overexpressing TRIP13 mutants. Student’s t -test with s.e.m. ; P <0.02. ( e ) Expression of mutant or wild-type Flag-tagged TRIP13 in stably expressing UM-SCC-1 cells was verified with anti-TRIP13 and anti-GAPDH antibodies. ( f ) A malachite green ATPase activity assay was performed with these cells. Student’s t -test with s.e.m. ; P <0.05. ( g ) A proliferation assay was performed with UM-SCC-1 cells stably overexpressing mutant or wild-type TRIP13 proteins along with control pCMV6 empty vector. Student’s t -test with s.e.m. ; P <0.04. ( h ) UM-SCC-1 cells stably expressing wild-type or mutant TRIP13 or control cells (pCMV6) were immunoblotted with anti-γH2AX, anti-actin antibodies and quantified (DU). ( i ) Mixed clonal population of UM-SCC-1 cells stably expressing wild-type or mutant TRIP13 or control cells were placed (1 × 10 6 cells each) on the CAM ( n =20, 5 in each group: two independent experiments). After incubating for 7 days, the upper CAM was excised and photographed (bar=5 mm). ( j ) The tumours (dotted boundary line) were measured and tumour volume was calculated. Student’s t -test with s.e.m. ; P <0.01 (* indicates statistically significant with corresponding P values). Full size image Chemotherapy and radiation are current treatment options for advanced SCCHN [31] . Resistance to treatment is correlated with recurrence and morbidity, underscoring the importance of developing new treatment strategies. Here we report that TRIP13 sensitizes SCCHN to a DNA-PKcs inhibitor. TRIP13 was designated as an oncogene by meta-analysis of several gene expression data sets and functionally validated as an oncogene by malignant transformation of non-malignant cells, tumour growth and invasion assays. Several NHEJ proteins were identified as binding partners of TRIP13, suggesting a role for TRIP13 in NHEJ, which was verified by multiple robust approaches. Consistent with the correlation between NHEJ and treatment resistance [27] , SCCHN cells overexpressing TRIP13 are resistant to chemotherapy and radiation but responsive to NHEJ inhibitors. Our studies define a mechanism of treatment resistance in cancer and emphasize the importance of targeting NHEJ to overcome treatment resistance in SCCHN overexpressing TRIP13. TRIP13 has not been investigated as an oncogene, although it is overexpressed in multiple cancers [32] , [33] , [34] , [35] . The TRIP13 gene is amplified in early-stage non-small cell lung cancer [33] . In a comparative genomic hybridization screen of 19 tumours, TRIP13 amplification was identified in 68% of tumours. We observed amplification of TRIP13 using FISH in ~15% of SCCHN, suggesting additional regulatory mechanisms. Using a bioinformatics approach, increased TRIP13 transcript and protein correlated with prostate cancer progression [36] . Another study reported overexpression of TRIP13 in a cutaneous lymphoma [37] . Before our study, the oncogenic role of TRIP13 had not been investigated. Although TRIP13’s function was unknown in humans, it has been investigated in mice, yeast and worms. In mice, TRIP13 is essential for non-crossover recombination during DSB repair but not at synaptic checkpoints during meiosis [10] , [38] , [39] . DSB repair occurs primarily via HR in germ cells and via NHEJ in somatic cells [40] . Our studies strongly support a role for TRIP13 in DSB repair via NHEJ. Previous studies showed that the role of TRIP13 varies between species. In yeast, worms and Drosophila melanogaster , Pch2 , the TRIP13 orthologue, is part of the synapsis checkpoint in germ cells [7] , [8] , [41] . In yeast, Pch2 is required for checkpoint arrest during defective recombination and synapsis [42] . Spermatocyte and oocyte death are observed in pachynema and birth in TRIP13 mutant mice. Although spermatocytes synapse completely, there is an accumulation of Rad51 (ref. 10 ). A recent network analysis of protein–protein interactions in mitosis suggested that TRIP13 is a kinetochore protein that interacts with the mitotic spindle but this was not experimentally verified [35] . Our data in SCCHN establish a role for TRIP13 in NHEJ. In humans, TRIP13 is located at chromosome 5p15 and encodes a protein of 432 amino acids. TRIP13 belongs to the AAA+ATPase family of chaperone proteins that facilitate assembly or degradation of protein complexes that regulate diverse cellular functions [22] . Hence, we investigated the binding partners of TRIP13 and identified the association of TRIP13 with repair proteins including KU70, KU80 and DNA-PKcs. During NHEJ, KU70 and KU80 form a heterodimer at the free DNA ends and recruit and activate DNA-PKcs, the catalytic subunit of DNA-dependent protein kinase [43] . Other members subsequently recruited to this DNA-PK complex include artemis, XRCC4 and DNA ligase IV. Our data also support the functional effect of TRIP13 ATPase activity. Given its role as an ATPase, it is possible that TRIP13 provides the energy needed for assembly of the DNA-PKcs complex. Future studies will elucidate this possibility. The DNA-PK complex may inhibit or promote apoptosis depending on the interacting proteins. Hence, regulation by proteins that are not part of the complex needs elucidation [20] . Together, our findings suggest a role for TRIP13 in cell survival via enhanced NHEJ. HR is error-free and essential for accurate transmission of genetic information. In contrast, NHEJ is error-prone, leading to mutations and cancer [6] . In our study, downregulation of TRIP13 led to a small increase of HR in BRCA1-deficient cells, likely because of functional BRCA2 in these cells. BRCA2, although not the primary transporter of RAD51, can bind and transport RAD51 to facilitate HR [44] . Radiation and chemotherapy, standard treatments for advanced SCCHN, promote apoptosis by inducing DSBs. Owing to minimal improvement in patient survival in five decades, the emphasis has moved to dose escalation. However, toxic effects on patients limit the extent to which radiation and chemotherapy can be intensified. Disruption of NHEJ promotes treatment sensitivity (apoptosis), whereas robust repair mediates treatment resistance (cell survival) [45] , [46] and poor clinical outcome. Moreover, since NHEJ occurs without a DNA template, chromosomal aberrations develop. Therefore, treatment that induces DSBs in cells with robust NHEJ leads to secondary malignancies, further decreasing patient survival [47] . In fact, a recent study showed that overexpression of Ku80 correlated with treatment failure and poor survival in SCCHN patients [48] . Hence, inhibitors of NHEJ could improve patient survival. In the present study, we showed that knockdown of TRIP13 sensitizes SCCHN cells to radiation and chemotherapy. Moreover, TRIP13 sensitizes cells to the DNA-PKcs’ inhibitor Nu7026. These findings suggest a therapeutic strategy in tumors overexpressing TRIP13 ( Fig. 9 ). 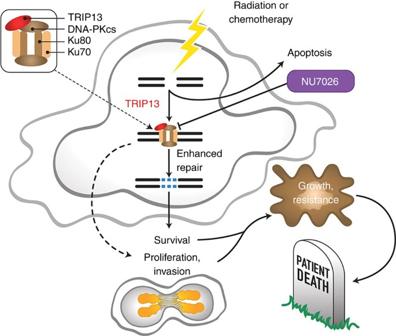Figure 9: Proposed mechanism for TRIP13-mediated treatment resistance via enhanced DNA repair. In the presence of TRIP13, treatment-induced DSBs are robustly repaired via NHEJ leading to cell survival (treatment resistance) and poor patient outcome in SCCHN. Tumours overexpressing TRIP13 are sensitive to NHEJ inhibitors (Nu7026). Figure 9: Proposed mechanism for TRIP13-mediated treatment resistance via enhanced DNA repair. In the presence of TRIP13, treatment-induced DSBs are robustly repaired via NHEJ leading to cell survival (treatment resistance) and poor patient outcome in SCCHN. Tumours overexpressing TRIP13 are sensitive to NHEJ inhibitors (Nu7026). Full size image Cisplatin–DNA adducts inhibit DNA-PKcs’ activity. TRIP13 overcomes this inhibition to promote NHEJ repair of DSBs by facilitating formation of the DNA-PKcs complex at the site of the break. Therefore, inhibition of TRIP13 in these tumours will sensitize them to the impact of cisplatin. Moreover TRIP13 overexpression induces DNA-PKCs phosphorylation (Ser2056) ( Supplementary Fig. 8B ) and may play a critical role in combined therapies bypassing HR repair. Cisplatin induces DNA-interstrand crosslinks, which induce single-strand breaks that are typically repaired by nucleotide excision repair. An important step in the repair of these crosslinks is DSBs. The lethality of cisplatin is reduced by efficient repair of DSBs by mechanisms such as NHEJ. Our data support that TRIP13 mediates DSB repair even when the HR is intact ( Fig. 6h ), that is, TRIP13 essentially hijacks repair to the NHEJ pathway. HR occurs during or immediately after DNA replication, in the S and G2 phases of the cell cycle when a template is available for repair. If the template is badly damaged or unavailable, HR repair cannot occur and the cell dies [45] , [46] . In this study we showed that TRIP13 mediates classical NHEJ, that is, a prominent repair pathway in mammalian cells that is active throughout the cell cycle [49] . DSB repair may also occur via the alternative NHEJ (aNHEJ) or microhomology-mediated end joining pathway that was described more recently [50] , [51] . The role of TRIP13, if any, in the aNHEJ pathway was not investigated. Although initial studies suggested that aNHEJ occurs when classical NHEJ is deficient, more recent studies show that aNHEJ occurs even in cells with competent classical NHEJ [49] . In contrast to classical NHEJ, aNHEJ is infrequent and does not require Ku70, Ku80 and DNA-PKcs [49] . In this study, we showed that TRIP13 binds to proteins in this DNA-PK complex and facilitates DSB repair in SCCHN. Thus, these studies define a new mechanism of treatment resistance and underscore the importance of targeting NHEJ to overcome treatment failure in SCCHN. Given the overexpression of TRIP13 in several treatment-resistant cancers, this strategy will likely be important for multiple cancers. Oncomine database Meta-analysis of TRIP13 in multiple cancers was performed using Oncomine ( http://Oncomine.org ) for SCCHN data sets and was graphed. Data sets used for this study were Cromer-Head-Neck [12] , Estilo-Head-Neck [13] , Ye-Head-Neck [14] , Kuriakose-Head-Neck [15] , Ginos-Head-Neck [16] and Toruner-Head-Neck [17] . Cell culture SCCHN cell lines were cultured as described [52] . All UM-SCC cell lines were provided by T. Carey (University of Michigan), and OSCC3 was provided by P. Polverini (University of Michigan). Cell lines were genotyped by the Sequencing Core at the University of Michigan pre- and post completion of studies. Genotype was verified against published sequences for UM-SCC cell lines [53] and OSCC3 was compared with an early passage (P2) of cells from source vial. OSCC3 cells were thought to be derived from a squamous cell carcinoma of the ventral tongue [54] , [55] ; however, HeLa cell contamination was recently identified [56] . Therefore, these cells may not be a pure SCCHN cell line. In this study, multiple cell lines and complementary approaches in different cell lines were used to elucidate the overall function of TRIP13. Primary oral keratinocytes were cultured according to the supplier’s instructions (ScienCell Research Laboratories, Carlsbad, CA, USA). NIH 3T3 cells were cultured in DMEM with 5% calf serum. HCC1937 cells were cultured in RPMI medium (Gibco no. 11875) with 10% fetal bovine serum (FBS; Gibco, no. 16000) and 1% Penicillin and streptomycin. COS-1 cells were cultured in DMEM (Gibco, no. 11965) with 10% FBS supplemented with penicillin and streptomycin. Q-RT–PCR Human oral keratinocytes (HOK), immortalized HOKs (HOK16B) and UM-SCC cell lines were grown to ~60% confluence and total RNA including microRNA was isolated using miRNAeasy kit (Qiagen, Valencia, CA, USA). cDNA was synthesized from total RNA using SuperScript III (Invitrogen, Carlsbad, CA). Quantitative real-time PCR was performed with Power SYBR Green Master Mix on an Applied Biosystems 7600HT Real Time PCR machine. Data were analysed by relative quantification method with normalization to GAPDH and then to normal keratinocytes. The forward and reverse primers were TRIP13GE-FP and TRIP13GE-RP, listed in the Supplementary Table 4 . Each sample was run in triplicate and the average fold change was determined. Immunoblot analysis Immunoblots were performed as described [57] , [58] . The primary antibodies were TRIP13 (1:3000, no. 19802-1-AP) from Proteintech, Chicago, IL, USA KU70 (1:1,000, no. AB1358), anti-phospho-H2AX(ser139) (γH2AX) (1:1,000, no. 05-636) both from Millipore, Billerica, MA, USA), KU80 (1:1,000, no. 2180), DNA-PKcs (1:1,000, no. 4602), anti-phospho-DNA-PKcs (Ser 2056) all from Cell Signaling Technology, Boston, MA, USA, and Actin (1:3,000, no. 612656) from BD Biosciences, Franklin Lakes, NJ, USA). Secondary antibodies were horseradish peroxidase (HRP)-conjugated goat anti-rabbit IgG or goat anti-mouse IgG (Jackson Immuno Research Laboratories, West Grove, PA, USA). For IP, TrueBlot secondary antibodies (eBioscience Rbt no. 18-8816, Mouse no. 18-8817) were used. Immunoreactive proteins were visualized using the SuperSignal-West-Pico-Chemiluminescent system (Pierce, Pittsburgh, PA, USA). The uncropped scanned films with molecular weight reference are included in the Supplementary Fig. 9 through 11 in sequence of appearance in the main text. Signal intensity was quantified using the ImageJ software ( http://rsbweb.nih.gov/ij/ ). Gene amplification (FISH) FISH hybridization was performed on genotyped SCCHN cell lines SCCHN TMA (US Biomax) using BAC clones (RP11-914L5-5′ clone; RP11-1040C13-3′ clone) for the TRIP13 break-apart probe. BAC clones were selected from UCSC genome browser and purchased through BACPAC resources (Children’s Hospital, Oakland, CA, USA). Fluorescence images were captured using a high-resolution CCD camera controlled using the ISIS image processing software (Metasystems, Germany). Immunohistochemistry Immunostaining on formalin-fixed, paraffin-embedded tissue and scoring of stain intensity was performed as described [59] on a SCCHN TMA (US Biomax). TRIP13 antibody for immunohistochemical studies was from Atlas Antibodies/Sigma Aldrich (Sigma, St Louis, MO, USA). Mouse IgG was used as negative control. For analysis of TMA data, interpretation and scoring were performed by a board-certified pathologist as described [58] . Multivariate analysis of TRIP13 activity was based on the Proportional Odds ordinal regression model. The analysis had intensity in the nucleus as the primary response variable, categorized as none, low, medium and high. Explanatory variables included cancer diagnosis (binary), TNM stage (ordinal, four categories), grade differentiation (ordinal, three categories), age (15–82) and gender (binary). Models were fit by maximizing the likelihood. Forward and stepwise variable selection procedures and the Likelihood Ration test were used to select the best model for the data and to test statistical hypotheses. Cell transfection and transduction TRIP13 was downregulated with TRIP13 siRNA (Dharmacon, Lafayette, CO, USA; sequence of siRNA used is listed in Supplementary Fig. 1C ). For overexpression of TRIP13, UM-SCC-1 cells were transfected with pCMV6-Flag-TRIP13 or pCMV6-Flag control vector (Origene, Rockville, MD, USA). For inducible TRIP13 downregulation, unique microRNA-30-based doxycycline-inducible Expression Arrest TRIPZ Lentiviral shRNAmir constructs were purchased from Thermo Scientific Open Biosystem. Two distinct TRIPZ oligonucleotide constructs in pTRIPZ vector (V2THS-28289, V3THS-345136) and control scrambled-shRNA were used to make lentiviral particles in the University of Michigan Vector-Core. After standardization, the lentiviral particles with V2THS-28289 were used for all experiments. Proliferation and invasion assays Cells were seeded at equal densities (2 × 10 4 for UM-SCC-22B, UM-SCC-5; and 1 × 10 4 for OSCC3 and COS-1) 24–48 h post transfection and counted at 1d, 3d and 5d. For CDDP-treated cells, 24–48 h after transfection cells were treated with CDDP or Nu7026 at the appropriate IC 50 for 2 h. Viable, nonviable and total cells were quantified with the Countess assay system using trypan blue (Invitrogen). Any P value, calculated using the Student’s t -test, less than 0.05 was accepted as significant. Cell invasion was assessed 24–48 h after transfection using the modified Boyden chamber assay with Transwell inserts (Corning, Lowell, MA, USA) coated with Matrigel (BD Biosciences), as described [52] . Control inserts, not coated with matrigel, were used as a control for migration. Any P value, calculated using the Student’s t -test, less than 0.05 was accepted as significant. Apoptosis Apoptosis was measured using flow cytometry [60] as well as TUNEL. For flow cytometry, cells were double-stained with fluorescein isothiocyanate (FITC)-labelled AnnexinV and PI using the FITC-AnnexinV Apoptosis Detection system (BD Biosciences). For detection of DNA strand breaks, nicks in DNA were labelled with the DeadEnd Fluorometric TUNEL kit (Promega, Madison, WI, USA) according to the manufacturer’s instructions. Formalin-fixed, paraffin-embedded tissue from in vivo experiments were analysed for apoptosis using TUNEL assay and the percent of FITC-positive cells was calculated. Cell cycle analysis Synchronized cells were dislodged with enzyme-free cell dissociation buffer (Invitrogen), centrifuged at 500 g at 4 °C, washed once in phosphate-buffered saline (PBS) and counted and were resuspended at one million per 500 μl ice-cold PBS and 4.5 ml of ice-cold 70% ethanol was added drop wise. Cells were then stored overnight at −20 °C. Cells were centrifuged and washed once with PBS, stained with 20 μg ml −1 PI (Sigma) in PBS containing 0.1% Triton X-100 and 200 μg ml −1 DNase-free RNaseA (Invitrogen) for 20 min at room temperature and analysed using flow cytometry. The DNA content ratio between G1 and G2 was calculated as 1.83 and used throughout each experiment. In vivo mouse xenograft model Stable inducible UM-SCC-22B-shTRIP13 as well as shcontrol cells were injected subcutaneously at bilateral sites in athymic nude mice (Ncr-nu/nu, age 4–6 weeks, male, n =10, 5 for each of the No-Dox- and Dox-treated group) at 1 × 10 6 cells per left and right sides of the back of the mice, respectively, according to the University of Michigan University Committee on Use and Care of Animals (UCUCA)-approved protocol [52] . Tumours were grown for 7 days. After 8d, five mice were administered normal water with 10% sucrose and the other five mice were given water containing 10% sucrose supplemented with 2 mg ml −1 doxycycline. Tumours were monitored and measured daily. A linear mixed effects statistical model was used to analyse the data. A random mouse-specific intercept term was included to adjust for tumour size measurements made on xenografts in the same mouse. Model-based Wald tests were used and a P value <0.05 was considered to be significant. In the TRIP13 overexpression study, stably overexpressing UM-SCC-1-TRIP13 and control cells (2 × 10 6 cells per site of each cell type) were injected subcutaneously at bilateral sites in athymic nude mice (Ncr-nu/nu, age 4–6 weeks, male, n =10, five in each group). Focus formation NIH3T3 cells were transfected using Lipofectamine 2000 (Invitrogen). After 72 h, cells were replated at ~1,000 cells per 60-mm plate and grown for 10 days. After fixing and washing with PBS, cells were stained with 0.2% crystal violet solution prepared in 70% ethanol. Foci were counted for each plate. CAM assay The CAM assay was performed as described [28] . Briefly, 3T3 cells stably expressing TRIP13 or control vector were seeded on the CAM of d10 chick embryos and incubated for 3 days. The CAMs were excised, sectioned and stained with haematoxylin and eosin. Invasive islands were quantified from multiple fields and graphed after normalization to control vector. Similarly, UM-SCC-1-TRIP13, TRIP13 mutants and control pCMV6 cells were seeded on the top of the CAM whenever needed and were treated with NU7026 after 24 h. P values were calculated using the Student’s t -test and any P value less than 0.05 was considered significant. Migration assay Cells were plated at 95% density in triplicate. Twenty-four hours later, cells were serum-starved for 6 h, and then treated with 25 mM of mitomycin C (Sigma) for 2 h in serum-free conditions. Media was removed and a scratch was made with a 200-μl pipette tip. Immediately after the scratch, complete media with 25 mM mitomycin C was added. Three fields in each replicate were photographed at 0=and=24 h. The area between the migration fronts was determined using the ImagePro Plus 5.1 (Media Cybernetics Inc, Bethesda, MD, USA) and the percentage migration at 24 h was calculated. Clonogenic assay Cells were irradiated at varying doses 24 h post seeding and colonies were grown for 7d–14d. After the appearance of colonies, cells were fixed with methanol containing crystal violet and quantified as described [61] . DNA fragmentation DNA was isolated from cells 4 h post radiation using PureLink Genomic DNA Mini Kit (Invitrogen). DNA fragmentation was visualized using agarose gel electrophoresis stained with ethidium bromide. Detection of DSBs Whole-cell lysates were collected from the cells irradiated with 2 Gy of IR at varying time points. Lysates were immunoblotted with γH2AX antibody and actin was as a loading control. Signal intensity was quantified and graphed over time. The number of γH2AX foci per cell was quantified in five fields in both NonTarget and siTRIP13. The average number of foci per cell was calculated and graphed. The Student’s t -test was used to calculate a P value. A P value less than 0.05 was accepted as significant. Comet assay Neutral comet assay was performed with treated cells. Glass slides with embedded cells in agarose were lysed in buffer containing 2.25 M sodium chloride, 8.9 mM Tris-HCl, 10% dimethylsulphoxide and 1% Triton X100 (pH=10) for 16 h. Lysed cells were equilibrated in running buffer TBE, electrophoresed and stained with Hoechst (Hoechst 33342, Invitrogen). After acquisition of images, the comet tail moment was analysed using the CometScore programme. Protein purification and mass spectrometry UM-SCC-1-FLAG-TRIP13 cells were used for TRIP13 protein purification by anti-Flag-M2 affinity gel (Sigma, no. A2220) and Flag-tagged protein was eluted with flag peptide. Lanes corresponding to control and TRIP13-flag were cut into 15 slices and destained with 30% methanol for 4 h. Upon reduction (10 mM dithiothreitol (DTT)) and alkylation (65 mM 2-chloroacetamide) of the cysteines, proteins were digested overnight with sequencing grade-modified trypsin (Promega). Resulting peptides were resolved on a nanocapillary reverse phase column (Picofrit Column, New Objective, Woburn, MA) using 1% acetic acid/acetonitrile gradient at 300 nl min −1 and directly introduced into a linear ion-trap mass spectrometer (LTQ Orbitrap XL, ThermoFisher Scientific, Rockford, IL, USA). Data-dependent MS/MS spectra on the five most intense ions from each full MS scan were collected (relative CE ~35%). Proteins were identified by searching the data against UniProt Human database appended with decoy (reverse) sequences using X!Tandem/Trans-Proteomic Pipeline software suite. All peptides and proteins with a peotideProphet and ProteinProphet probability score of >0.9 (fdr<2%) were considered positive identifications. Proteins found in the control lane were subtracted using in-house subtraction programme and the remaining were considered as potential interactors. Co-immunoprecipitation Immunoprecipitation of TRIP13 co-complex proteins was performed by Pierce Co-IP kit (ThermoFisher Scientific, no. 26149). DSB repair assay DNA DSB-repair assays were performed using chromosomally integrated reporter constructs for both HR or NHEJ [26] . Plasmids containing the HR or NHEJ cassettes were linearized by digesting with NheI endonuclease (New England BioLabs, Ipswich, MA, USA) and gel-purified using Qiagen gel extraction kit (Cat no. 28704). One microgram of this plasmid was used to transfect HR-deficient (BRCA1-mutant) cells, HCC1937, using the amaxa kit (Lonza, Allendale, NJ, USA) with the U20 programme. Cells were selected with G418 and maintained in the presence of 250 μg of G418 in RPMI media containing 10% FBS and 1% penicillin/streptomycin. HCC1937 cells stably transfected with HR or NHEJ cassettes were transfected with NT or siTrip13 siRNAs. Forty-eight hours after transfection DSBs were induced by transfecting cells with 5 μg I-SceI expression plasmid using the Amaxa kit, U20 programme with 0.1 μg of dsRed expression plasmid as transfection control. Three days after transfection, cells were analysed using flow cytometry for efficiency of DSB repair. GFP and dsRed expression plasmids were used as controls. The ratio of dsRed/GFP was calculated to represent the amount of DNA repair occurring. The Student’s t -test was used to calculate P values. A P value less than 0.05 was accepted as significant. End joining assay Mini NHEJ–whole cell extract (mNHEJ–WCE) preparation and in vitro end joining experiment were carried out according to Smeaton et al . [62] Briefly, cells were grown to 70–80% confluency after appropriate treatment and were collected by scraping in PBS. Cells were washed twice in PBS, pelleted and snap-frozen on dry ice. Frozen cell pellets were resuspended in 2 packed cell volumes of hypotonic lysis buffer (10 mM Tris (pH 8), 1 mM EDTA (pH 8), 5 mM DTT) and incubated on ice for 20 min with repeated vortexing. Cells were centrifuged for 2 min at 800 g and the supernatant was collected and stored on ice. The pellet was resuspended in 1 packed cell volume of nuclear extract buffer (25 mM Tris (pH 8), 1.5 mM EDTA (pH 8), 330 mM KCL) and incubated on ice for 20 min. Retained supernatant was added back, re-suspended well and centrifuged for 10 min at 16,500 g at 4 °C. The supernatant (mNHEJ–WCE) was quantified for total protein, adjusted for concentration and stored in small aliquots at −80 °C after quick freezing in liquid nitrogen. Approximately 250 ng of gel-purified pcDNA3.1 plasmid double-digested with Xho I/ Bam HI (to generate noncohesive end) was incubated with 25 μg (5 μl) of mNHEJ–WCE, and 0.25 units of T4 ligase as positive control in 50 mM Tris (pH 7.5),10 mM MgCl 2, 10 mM DTT, 1 mM ATP, in a reaction volume of 25 μl. The reaction was incubated at 37 °C for 1 h. The reaction was stopped by adding 2.5 μl of 0.5 M EDTA and 2.5 μl of 10% SDS. DNA was purified using the Qiagen PCR purification Kit and loaded on a 0.8% agarose gel, stained with ethidium bromide. Recircularized DNA was visualized and photographed. γH2AX and Rad51 colocalization using immunofluorescence Cells were stained with RAD51 (1:500) and γH2AX antibody (1:1,000) in 0.3% triton X-100 overnight at 4 °C. Cells were washed and incubated with secondary antibodies sequentially and imaged on an Olympus BX-51 microscope at the Microscopy and Image Analysis Core (University of Michigan). The number of colocalized foci (orange) per cell was quantified from five fields of cells in both NonTarget and siTRIP13. The average number of foci per cell was graphed. The Student t -test was used to calculate a P value. A P value <0.05 was accepted as significant. Half maximal inhibitory concentration (IC 50 ) Cells were seeded at ~1 × 10 4 cells per well. For CDDP, cells were treated with varying concentrations ranging from 0 to 30 μM, in triplicate for 2 h. Cells were counted 72 h later. Each concentration was graphed as a percent of control (0 μM) and the dose at which only 50% of the cells survived was calculated. For NU7026, cells were treated with varying concentrations ranging from 0 to 15 μM in triplicate for 72 h. Each concentration was presented in a graph as a percent of the control (0 μM) and the dose at which only 50% of the cells survived was calculated. TRIP13 mutant construct TRIP13-WalkerA (TRIP13 G184A ) mutant was generated using site-directed mutagenesis of the conserved WalkerA motif of TRIP13 at the region of (179) G PPGT GK T(186) using primers TRIP13WALKERAG184ASe and TRIP13WALKERAG184AAs. The two PCR fragments were generated using wild-type TRIP13-cDNA as template and first primer set TRIPFullCloneOriFP and TRIP13WALKERAG184AAs and with second primer set TRIP13WALKERAG184ASe and TRIPFullCloneOriRP. PCR conditions were 95 °C for 4 min, 55 °C for 1 min followed by 30 cycles of 95 °C for 30 s, 55 °C for 30 s, 70 °C for 1 min and two hold at 70 °C for 6 min and at 4 °C forever. The PCR fragments were gel-purified and used for a second PCR using equal molar ratios of each fragment and with two end primers, TRIPFullCloneOriFP and TRIPFullCloneOriRP. The PCR conditions were: 95 °C for 6 min, 55 °C for 6 min followed by 12 cycles of 95 °C for 30 s, 55 °C for 30 s, 70 °C for 1 min and two hold at 70 °C for 6 min and at 4 °C forever. The final full fragment was gel-purified, double-digested with BamHI and XhoI and ligated to the pCMV6 vector. Similarly, theTRIP13 deletion mutant was generated by deleting 20 conserved amino acids (293–312) from the ATPase domain of TRIP13 using primers TRIP13AAADelFP and TRIP13AAADelRP with similar PCR conditions. All primers are listed in the Supplementary Table T4 . The PCR amplification was performed with Hi-fidelity Taq polymerase (Invitrogen no. 11304-011). Malachite green ATPase assay Malachite green assay was performed according to Lanzetta et al . [63] for ATPase activity of wild-type TRIP13 and mutant proteins. Malachite green dye was prepared by combining 30 ml of 0.045% of Malachite green dye (Sigma no. 38800) in H 2 O and 10 ml of 4.2% ammonium molybdate (Sigma no. A1343) in 4N HCl (Fisher no. SA56-1) and 800 μl of 1% Triton X-100. The dye was left at room temperature in dark for 1 h and filtered through a 0.45-μm filter (Millipore no. SLHA033SS). The dye was prepared freshly every time before the experiment. Citric acid (34%) was prepared in H 2 O and filtered. One million of each control cells and cells overexpressing TRIP13 or mutant proteins in either transiently transfected in COS-1 cells or stably transfected in UM-SCC-1 cells were lysed in 392 μl of buffer containing 50 mM Triethanolamine (TEA), 50 mM KCl, 20 mM MgCl 2 (pH 7.5) and 6 mM CHAPS and incubated on ice for 5 min with repeated brief vortexing. At the end of the incubation, 8 μl of 100 mM ATP was added (final 2 mM) and mixed thoroughly. Fifty microlitres of this mixture were added immediately (0 time point) to 400 μl of malachite green dye solution and incubated at room temperature for 1 min and stopped with 100 μl of 34% citric acid and absorbance ( A 660 ) was measured. Subsequent measurements were taken at 2-min intervals till 12 min. Background was eliminated by subtracting A 660 value from each with a blank absorbance with dye and the buffer. The protein content of cell lysates was quantified and ATPase activity was normalized per microgram of protein. Each experiment was performed three times with three replicates within each experiment. How to cite this article: Banerjee, R. et al . TRIP13 promotes error-prone nonhomologous end joining and induces chemoresistance in head and neck cancer. Nat. Commun. 5:4527 doi: 10.1038/ncomms5527 (2014).